Mesoscale infraslow spontaneous membrane potential fluctuations recapitulate high-frequency activity cortical motifs Neuroimaging of spontaneous, resting-state infraslow (<0.1 Hz) brain activity has been used to reveal the regional functional organization of the brain and may lead to the identification of novel biomarkers of neurological disease. However, these imaging studies generally rely on indirect measures of neuronal activity and the nature of the neuronal activity correlate remains unclear. Here we show, using wide-field, voltage-sensitive dye imaging, the mesoscale spatiotemporal structure and pharmacological dependence of spontaneous, infraslow cortical activity in anaesthetized and awake mice. Spontaneous infraslow activity is regionally distinct, correlates with electroencephalography and local field potential recordings, and shows bilateral symmetry between cortical hemispheres. Infraslow activity is attenuated and its functional structure abolished after treatment with voltage-gated sodium channel and glutamate receptor antagonists. Correlation analysis reveals patterns of infraslow regional connectivity that are analogous to cortical motifs observed from higher-frequency spontaneous activity and reflect the underlying framework of intracortical axonal projections. The brain exists in a state of constant activity. This activity occupies a wide temporal landscape encompassing a frequency range spanning many orders of magnitude from hundreds to hundredths of Hertz [1] . Although much is known about the determinants and function of higher-frequency activity, less is known about very low-frequency forms of activity (<0.1 Hz). These questions are of particular importance as the physiological role and exploitation of very low-frequency spontaneous or resting-state activity have become the subjects of substantial and intense interest given that these frequencies are typically resolved using functional magnetic resonance imaging (fMRI) [2] , [3] . From its early description as ‘infraslow’ [4] , spontaneous or resting-state activity at this very low-frequency domain (<0.1 Hz) has been observed as a consistent feature of ongoing brain activity across different species [4] , [5] , [6] , [7] and across different brain states [5] , [8] , [9] , [10] , though its precise function and mechanistic underpinnings remain unclear. In the developing brain, electrophysiological infraslow activity in the form of neuronal activity transients or bursting activity has been linked with the development of neuronal networks [11] , [12] , whereas in the adult brain, infraslow activity has been demonstrated to synchronize with higher-frequency brain activity [13] , [14] and to correlate to variability in behavioural performance [15] , [16] . Renewed focus on the nature of spontaneous resting-state infraslow activity has been precipitated due to an immense proliferation of functional neuroimaging studies that have revealed much about the brain’s functional organization and have identified what has been described as the brain’s Default Mode Network (DMN) [17] , a network of brain structures that are coherently, highly active at rest and reduced during active task performance [18] . The DMN may represent a consistent functional organizing principle and infraslow spontaneous activity of this kind may play a profound role in modulating and/or synchronizing higher-frequency brain activity due to cross-frequency, phase–amplitude coupling [10] , [13] , [14] . Furthermore, alterations in its structure have been linked with neurodegenerative and psychiatric disease [19] , [20] , [21] suggesting the potential for the identification of novel biomarkers and a greater understanding of both disease progression and recovery. Because neuroimaging studies of infraslow functional connectivity are dominated by fMRI which reports on a surrogate signal of neuronal activity, blood oxygen level dependent (BOLD) contrast, the interpretation of the underlying neurophysiology is indirect and nuanced [22] , particularly, in light of evidence illustrating instances of dissociation between neuronal activity and hemodynamic responses [23] , [24] , [25] , [26] such as ipsilateral or non-crossed sensory responses where increases in neuronal activity are followed by reductions in blood flow [26] . Furthermore, the temporal resolution of fMRI is limited and questions of the underlying neuronal activity correlate cannot be directly assessed by these means. In this work, we used high-speed, wide-field, voltage-sensitive dye (VSD) imaging to investigate the presence and functional structure of infraslow spontaneous activity in anaesthetized and awake mouse cortex. This imaging paradigm is ideally suited for this study as VSD imaging directly reflects underlying electrical activity with high spatial and temporal resolution allowing for imaging of nearly the entire dorsal neocortex while maintaining high spatial resolution and at rates sufficient to resolve multiple time signatures of ongoing activity. The signal is dependent on neuronal activity [27] and the red spectral properties of the dye [28] mitigate potentially confounding neuroimaging artifacts such as flavoprotein autofluorescence, intrinsic signal responses, and heartbeat and respiration artifacts [28] , [29] . Such confounding artifacts are potentially present in all the signals attributed to green epifluorescence (including genetically encoded Ca 2+ indicators). We demonstrate the presence of spontaneous infraslow activity in anaesthetized mouse cortex and that this activity exhibits regionally selective patterns, correlates with independent measures of electroencephalography (EEG) and local field potential (LFP), and is bilaterally synchronous. Importantly, intrahemispheric, spontaneous infraslow activity exhibits a patterned regional structure that is analogous to cortical motifs within higher-frequency (0.5–6 Hz) activity that we have previously described [27] . This builds upon pioneering studies in cat visual cortex which illustrated that cortical orientation representations are dynamically represented in ongoing spontaneous activity, and further, that these events may serve a preparatory role in setting default cortical sensory input parameters [30] , [31] . Local and global infraslow activity in anaesthetized mouse We simultaneously recorded spontaneous EEG signals using a direct current (DC) amplifier and LFP from a surface electrode placed near primary somatosensory cortex and from a glass micropipette inserted into layer 2/3, respectively, from urethane-anaesthetized mice ( Fig. 1a ). Anaesthesia via urethane provided a long-lasting, stable baseline brain state that was devoid of active behaviours and voluntary mental processes that may contaminate the analysis of purely spontaneous activity from which to make our observations. This is of critical importance in the analysis of infraslow activity given its, by definition, very slow nature and the consequently long-duration observation times necessary to assess it. Furthermore, descriptions of resting-state infraslow activity in humans, non-human primates and rodents have demonstrated these networks to be robust and persistent in task-negative awake states in addition to states of natural sleep and anaesthesia [5] , [9] , [32] . Furthermore, our previous data indicated that connectivity maps from quiet awake and anaesthetized states are similar [27] , [33] . We observed spontaneous infraslow (<0.1 Hz) fluctuations in baseline DC-EEG and LFP recordings ( Fig. 1a ). These fluctuations in baseline were accompanied by parallel spontaneous infraslow modulation of the power of higher-frequency activity suggesting a nested relationship with underlying infraslow activity ( Fig. 1b ). This modulation of higher-frequency activity was most evident in the delta frequency band (1.5–4 Hz; Fig. 1c ). The power spectra of EEG recordings revealed a broad peak centred at 1 Hz consistent with the presence of activity associated with slow oscillations ( Fig. 1d ) [34] . Interestingly, we also note the presence of substantial signal power in the infraslow frequency range (<0.1 Hz). This activity lacked the fully resolved structure of a local peak in the power spectrum that typically signifies truly oscillatory activity and thus has been interpreted as underlying low-frequency asynchronous brain activity [2] , [10] , [14] . We quantified infraslow EEG signal power across an infraslow frequency range (0.009–0.08 Hz) typically associated with brain activity used in functional connectivity analyses of resting-state functional magnetic resonance imaging (fc-fMRI) studies [18] , [35] ( Fig. 1d ). However, detrending the EEG spectrum [36] within the delta power band reveals infraslow fluctuations (0.009–0.08 Hz; Fig. 1d ; n =11 mice). Treatment of the cortex with topical local application of the voltage-gated sodium channel blocker, tetrodotoxin (TTX) or the glutamate receptor antagonists, 6,7-dinitroquinoxaline-2,3-dione (DNQX) and (2R)-amino-5-phosphonovaleric acid (AP5), resulted in a large attenuation of infraslow EEG power that was not observed when treated with the dimethyl sulfoxide (DMSO) vehicle control alone ( Fig. 1e ). These results indicated that the underlying basis of this activity relies upon cortical excitability and glutamatergic signalling and is not an artifact of systemic physiological parameter alterations or instrument noise. 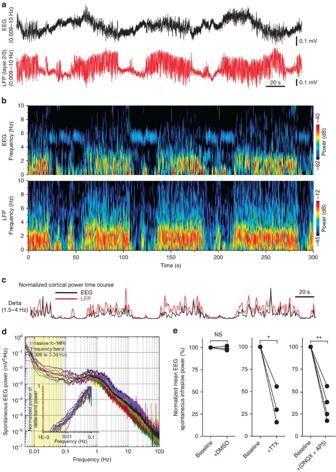Figure 1: Global and local infraslow fluctuations in spontaneous activity from mouse cortex. (a) Top (black trace), 5 min segment of DC acquired-EEG recording of spontaneous activity from an electrode placed near the surface of somatosensory cortex illustrating infraslow (<0.1 Hz) fluctuations in baseline activity and amplitude. Bottom (red trace), simultaneous recording of spontaneous activity from an LFP electrode inserted into layer 2/3 of somatosensory cortex. Both signals were filtered offline at 0.009–10 Hz for presentation. (b) Spectrograms of EEG and LFP recordings ina(0.1–200 Hz bandpass filtered) illustrating infraslow power modulation of low-frequency activity. (c) Normalized cortical power time course (delta frequency 1.5–4 Hz) of EEG and LFP signals ina. (d) Raw power spectrum of spontaneous DC-EEG activity in 15-min recordings from 10 individual anaesthetized mice plotted on log–log axes. Black line denotes the average of the individual power spectra. Shaded yellow region denotes frequency band of activity associated with fc-fMRI. Inset, detrending spectrum analysis illustrating power spectra of integrated delta power time series for each individual animal. Note, power fluctuations within the infraslow frequency band (0.009–0.08 Hz). (e) Normalized mean EEG power from the fc-fMRI infraslow frequency band (0.009 to 0.08 Hz) recorded before (baseline) and after topical, cortical surface application of vehicle control (0.4% DMSO,n=3), TTX (10 μM,n=3), or combined DNQX (200 μM) and AP5 (500 μM,n=3). *P<0.05 and **P<0.01, pair-samplet-test. Figure 1: Global and local infraslow fluctuations in spontaneous activity from mouse cortex. ( a ) Top (black trace), 5 min segment of DC acquired-EEG recording of spontaneous activity from an electrode placed near the surface of somatosensory cortex illustrating infraslow (<0.1 Hz) fluctuations in baseline activity and amplitude. Bottom (red trace), simultaneous recording of spontaneous activity from an LFP electrode inserted into layer 2/3 of somatosensory cortex. Both signals were filtered offline at 0.009–10 Hz for presentation. ( b ) Spectrograms of EEG and LFP recordings in a (0.1–200 Hz bandpass filtered) illustrating infraslow power modulation of low-frequency activity. ( c ) Normalized cortical power time course (delta frequency 1.5–4 Hz) of EEG and LFP signals in a . ( d ) Raw power spectrum of spontaneous DC-EEG activity in 15-min recordings from 10 individual anaesthetized mice plotted on log–log axes. Black line denotes the average of the individual power spectra. Shaded yellow region denotes frequency band of activity associated with fc-fMRI. Inset, detrending spectrum analysis illustrating power spectra of integrated delta power time series for each individual animal. Note, power fluctuations within the infraslow frequency band (0.009–0.08 Hz). ( e ) Normalized mean EEG power from the fc-fMRI infraslow frequency band (0.009 to 0.08 Hz) recorded before (baseline) and after topical, cortical surface application of vehicle control (0.4% DMSO, n =3), TTX (10 μM, n =3), or combined DNQX (200 μM) and AP5 (500 μM, n =3). * P <0.05 and ** P <0.01, pair-sample t -test. Full size image VSD imaging of spontaneous cortical infraslow activity We have characterized repeating structures resembling sensorimotor activity, which we have referred to as cortical motifs, within higher-frequency spontaneous activity in anaesthetized and quiet awake mice [27] . We used a similar strategy to investigate the spatiotemporal structure of spontaneous infraslow cortical activity and examine how this activity relates to our previously published observations. In agreement with our observed high power in the infraslow band arising from measurements of spontaneous activity using cortical EEG and LFP recordings, we investigated whether this signal was also reflected in our wide-field, voltage-sensitive dye imaging of spontaneous cortical activity ( Supplementary Fig. 1 ). We acquired continuous 30 min epochs of voltage-sensitive dye imaging of spontaneous activity from anaesthetized mice ( Fig. 2 ). Spontaneous activity was recorded in a quiet, dark, enclosed partition and in the absence of any external sensory stimulation. Red light used for VSD excitation was directed away from the eyes and illumination was kept constant during image acquisition to avoid intermittent stimulation. The time course of the raw VSD fluorescence signal decayed exponentially consistent with some degree of photobleaching ( Supplementary Fig. 1 ), however, the time course of both EEG power and the power of VSD fluorescence was steady for the duration of our recordings indicating both photostability of the dye and stability of the underlying brain state being sampled ( Supplementary Fig. 2 ). A broad local peak in the power spectra indicated oscillatory activity associated with the slow oscillation (1 Hz) [34] , [37] and delta oscillation (1.5–4 Hz), which predominate under anaesthesia and natural sleep and can be observed in states of quiet wakefulness [27] , [33] , [34] . As in our DC-EEG and LFP recordings of spontaneous activity, we observe the presence of substantial power in the infraslow frequency (<0.1 Hz) range indicating a significant presence of infraslow spontaneous activity in our cortical VSD signals ( Supplementary Fig. 1b ). 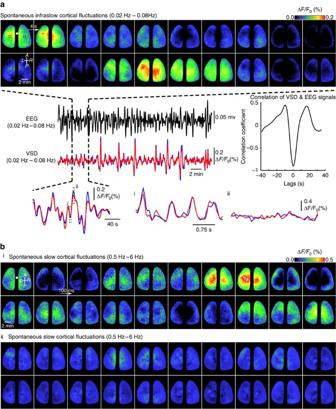Figure 2: Spatiotemporal characteristics of spontaneous, infraslow fluctuations revealed by voltage-sensitive dye imaging. (a) Montage of spontaneous, infraslow (0.02–0.08 Hz) bilateral VSD activity in cortex corresponding to the segment of time depicted by the dashed black lines to the EEG signal below. Successive image frames depict 4 s intervals. Blue and red dashed boxes indicate position of ROIs centred on the right (R)- and left (L)-HLS1, respectively. Images in montage have been scaled to the colour bar. Comparison of time courses of simultaneously acquired infraslow VSD signal measured from ROIs from L-HLS1 (blue) and R-HLS1 (red) with the EEG signal (black) of a closely positioned EEG electrode. Cross-correlogram depicting the cross-correlation of EEG and VSD signals. Expansion in time of infraslow VSD signals depicting time course of higher-frequency activity (0.5–6.0 Hz) at two phases of infraslow spontaneous activity (dashed black boxes denoted by i and ii). Compass arrows indicate anterior (A), posterior (P), left (L) and right (R) directions. White circle denotes the position of the bregma. (b) Montage of higher-frequency VSD spontaneous ‘up-down’ state activity (0.5 to 6.0 Hz) taken from a period of peak infraslow activity (a-i) and trough infraslow activity (a-ii). Images have been scaled to the depicted colour bar. Figure 2: Spatiotemporal characteristics of spontaneous, infraslow fluctuations revealed by voltage-sensitive dye imaging. ( a ) Montage of spontaneous, infraslow (0.02–0.08 Hz) bilateral VSD activity in cortex corresponding to the segment of time depicted by the dashed black lines to the EEG signal below. Successive image frames depict 4 s intervals. Blue and red dashed boxes indicate position of ROIs centred on the right (R)- and left (L)-HLS1, respectively. Images in montage have been scaled to the colour bar. Comparison of time courses of simultaneously acquired infraslow VSD signal measured from ROIs from L-HLS1 (blue) and R-HLS1 (red) with the EEG signal (black) of a closely positioned EEG electrode. Cross-correlogram depicting the cross-correlation of EEG and VSD signals. Expansion in time of infraslow VSD signals depicting time course of higher-frequency activity (0.5–6.0 Hz) at two phases of infraslow spontaneous activity (dashed black boxes denoted by i and ii). Compass arrows indicate anterior (A), posterior (P), left (L) and right (R) directions. White circle denotes the position of the bregma. ( b ) Montage of higher-frequency VSD spontaneous ‘up-down’ state activity (0.5 to 6.0 Hz) taken from a period of peak infraslow activity ( a- i) and trough infraslow activity ( a- ii). Images have been scaled to the depicted colour bar. Full size image Infraslow activity is regional and bilaterally synchronous To assess the spatiotemporal structure of specifically infraslow spontaneous activity, we down-sampled our acquired imaging data by integrating video frames to a sampling rate of 1 Hz and then applied a zero-phase lag Chebyshev bandpass (0.02–0.08 Hz) filter. This frequency band was selected on the basis of previous reports of infraslow activity in rodents and our own measurements of VSD signal power and functional structure [6] , [7] , [38] , [39] . We observed fluctuations in the resultant VSD signal ( Supplementary Fig. 1 ) and the observed power spectra indicated a >100,000-fold attenuation of signal power above 0.2 Hz ( Supplementary Fig. 1b ) giving us confidence that our VSD signal was reflecting truly infraslow activity. Using a giant, bilateral, cranial window experimental preparation [33] , [40] , [41] , we showed that infraslow spontaneous cortical activity exhibits bilaterally synchronous, regionally discrete areas of activation ( Fig. 2a and Supplementary Movie 1 ). VSD signal fluctuation time courses derived from left- and right-hemisphere hindlimb somatosensory (HLS1) representations were virtually identical. Cross-correlation of VSD HLS1 signal with simultaneously recorded EEG from a closely positioned surface electrode similarly exhibited high correlation ( Fig. 2a ). We next examined the presence of higher-frequency (0.5–6.0 Hz) activity that we have previously described [27] , [33] , herein referred to as ‘slow spontaneous activity’ to differentiate it from infraslow activity ( Supplementary Fig. 1 ), embedded within ongoing infraslow spontaneous activity. We found that in the slow spontaneous frequency band there were extended periods of high and low activity dependent on the phase of ongoing infraslow spontaneous activity ( Fig. 2b ). A systematic analysis of regional bilaterally synchronous infraslow spontaneous activity was examined. On the basis of individual, experimentally derived sensory stimulation-based mapping of functional cortical regions ( Supplementary Fig. 3 ) and extrapolated coordinates for non-sensorimotor regions from reference atlases, we selected 12 regions of interest (ROIs) and their homotopic representations in the contralateral hemisphere ( Fig. 3a ) and determined interhemispheric cross-correlation of infraslow spontaneous activity. We revealed a high degree of correlation across all examined regions of the cortex with the highest correlation exhibited by midline regions including the anterior segment of secondary motor cortex/anterior cingulate (aM2/AC), the posterior segment of secondary motor cortex (pM2) and retrosplenial (RS) cortex ( Fig. 3b ). Statistical comparison of clustered cortical regions in midline (aM2/AC, pM2, mBC and RS), somatomotor (FLS1, HLS1, mFL and mHL) and visual systems (V1 and V2MM and V2LM) confirmed these observations ( Fig. 3c ). 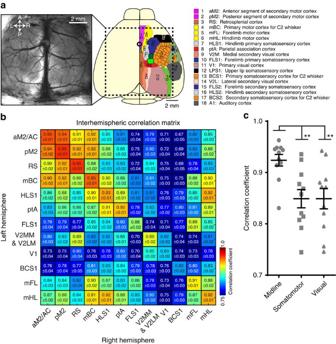Figure 3: Infraslow spontaneous activity interhemispheric regional correlation. (a) Cartoon schematic of the bilateral cranial window imaging field of view with the locations of cortical ROIs depicted: aM2/AC, anterior segment of secondary motor cortex/anterior cingulate; pM2, posterior segment of secondary motor cortex; RS, retrosplenial cortex; mBC, primary motor cortex for C2 whisker; HLS1, primary hindlimb somatosensory cortex; ptA, parietal association cortex; FLS1, primary forelimb somatosensory cortex; V2MM and V2LM, mediomedial and lateromedial secondary visual cortex; V1, primary visual cortex; BCS1, primary barrel cortex; mFL, forelimb motor cortex; mHL, hindlimb motor cortex. (b) Correlation matrix comparing the activity of 24 ROIs from the left and right hemispheres from 30 min of infraslow spontaneous activity illustrating a high degree of bilateral symmetry (n=11 mice). Correlations for each ROI are reported as mean±s.e.m. Correlation matrix is scaled to the indicated colour bar. (c) Cortical regions were grouped into left and right hemisphere midline (aM2/AC, pM2, mBC and RS), somatomotor (FLS1, HLS1, mFL, mHL) and visual systems (V1 and V2MM and V2LM) and the magnitude of bilateral correlation was compared (n=11 mice). Group means are depicted by horizontal lines. Error bars are s.e.m. ** denotesP<0.01 (one-way analysis of variance, Bonferronipost hoc). Figure 3: Infraslow spontaneous activity interhemispheric regional correlation. ( a ) Cartoon schematic of the bilateral cranial window imaging field of view with the locations of cortical ROIs depicted: aM2/AC, anterior segment of secondary motor cortex/anterior cingulate; pM2, posterior segment of secondary motor cortex; RS, retrosplenial cortex; mBC, primary motor cortex for C2 whisker; HLS1, primary hindlimb somatosensory cortex; ptA, parietal association cortex; FLS1, primary forelimb somatosensory cortex; V2MM and V2LM, mediomedial and lateromedial secondary visual cortex; V1, primary visual cortex; BCS1, primary barrel cortex; mFL, forelimb motor cortex; mHL, hindlimb motor cortex. ( b ) Correlation matrix comparing the activity of 24 ROIs from the left and right hemispheres from 30 min of infraslow spontaneous activity illustrating a high degree of bilateral symmetry ( n =11 mice). Correlations for each ROI are reported as mean±s.e.m. Correlation matrix is scaled to the indicated colour bar. ( c ) Cortical regions were grouped into left and right hemisphere midline (aM2/AC, pM2, mBC and RS), somatomotor (FLS1, HLS1, mFL, mHL) and visual systems (V1 and V2MM and V2LM) and the magnitude of bilateral correlation was compared ( n =11 mice). Group means are depicted by horizontal lines. Error bars are s.e.m. ** denotes P <0.01 (one-way analysis of variance, Bonferroni post hoc ). Full size image Infraslow cortical motifs We have previously implemented a seed pixel-based region-of-interest strategy that is widely used in fc-fMRI studies to generate correlation maps based on a seed pixel within a distinct cortical area to identify repeating patterns of activity, referred to as cortical motifs, within spontaneous activity in the frequency range of 0.5 to 6.0 Hz in anaesthetized and awake mice [27] . This frequency range of activity encompassed previously well-characterized activity of the slow oscillation as well as cortical delta activity both of which predominate under states of anaesthesia and in quiet wakefulness [27] , [33] . Using high-speed imaging, we acquired epochs of spontaneous cortical activity at high video sampling rates that allowed us to examine the spatiotemporal structure of spontaneous infraslow activity and directly compare it with our cortical motifs derived from slow activity for the same period ( Supplementary Movie 2 ). This permitted direct comparisons of cortical motif structures between the two activity bands that are internally controlled within an individual animal while also acting to control for potential external variables such as differing recording conditions, altered brain states, anaesthetic depth changes and photostability of the dye. Correlation maps generated from placing a seed pixel within a functionally defined cortical region, such as the forelimb primary somatosensory representation, FLS1, strongly resembled the correlation map generated from slow spontaneous activity, which we have previously described as reflecting the sensory-evoked patterns of activity of forelimb sensation ( Fig. 4a ). This similarity included features of distant, long-range, remote connectivity associated with secondary forelimb somatosensory cortices (FLS2) that were identified in both infraslow and slow spontaneous activity. Analogous correlation maps were computed for seed pixel locations in additional sensory cortices, hindlimb primary somatosensory (HLS1) and primary visual (V1) as well as the association cortices, retrosplenial cortex (RS) and parietal association cortex (ptA). We also tested the persistence of infraslow functional organization during awake states. We obtained spontaneous activity from mice during periods of quiet wakefulness and were able to demonstrate similar seed map-based functional organization within infraslow and slow spontaneous activity ( Fig. 4b ). As done previously [27] , a spatial correlation analysis of correlation maps derived from infraslow versus slow spontaneous activity was used to determine the significance of these similarities ( Fig. 4c and Supplementary Fig. 4 ). 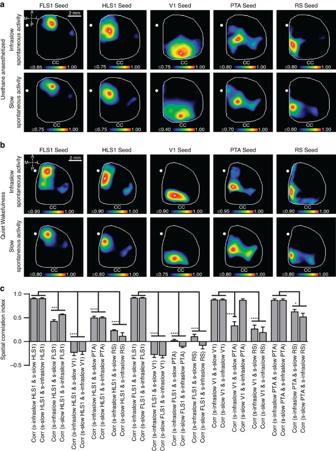Figure 4: Infraslow functional connectivity recapitulates connectivity observed in slow spontaneous activity. (a) Representative correlation maps generated from 30 min of infraslow (top) and slow frequency (bottom) spontaneous activity imaged through a unilateral cranial window for seed pixels located within primary forelimb somatosensory (FLS1), primary hindlimb somatosensory (HLS1), visual (V1), parietal association (PTA) and retrosplenial (RS) cortices. Correlation coefficient (CC) values for each map are scaled to the colour bar located immediately below. (b) As ina, representative correlation maps generated from 10–30 min of spontaneous activity derived from states of quiet wakefulness. (c) Statistical comparison of infraslow and slow frequency correlation maps generated from spontaneous, quiet awake activity inbby spatial correlation analysis (n=7). Error bars represent s.e.m. *, *** and **** denoteP<0.05,P<0.001 andP<0.0001, respectively (one-way analysis of variance, Bonferronipost hoc). Figure 4: Infraslow functional connectivity recapitulates connectivity observed in slow spontaneous activity. ( a ) Representative correlation maps generated from 30 min of infraslow (top) and slow frequency (bottom) spontaneous activity imaged through a unilateral cranial window for seed pixels located within primary forelimb somatosensory (FLS1), primary hindlimb somatosensory (HLS1), visual (V1), parietal association (PTA) and retrosplenial (RS) cortices. Correlation coefficient (CC) values for each map are scaled to the colour bar located immediately below. ( b ) As in a , representative correlation maps generated from 10–30 min of spontaneous activity derived from states of quiet wakefulness. ( c ) Statistical comparison of infraslow and slow frequency correlation maps generated from spontaneous, quiet awake activity in b by spatial correlation analysis ( n =7). Error bars represent s.e.m. *, *** and **** denote P <0.05, P <0.001 and P <0.0001, respectively (one-way analysis of variance, Bonferroni post hoc ). Full size image Given the susceptibility of infraslow frequency fluctuations to be potentially confounded by non-neuronal phenomenon, we examined the mechanistic basis underlying our observed infraslow fluctuations [7] , [42] , [43] , [44] . Topical treatment of the cortical surface with TTX (10 μM), a voltage-gated sodium channel antagonist, completely abolished whisker sensory stimulation-evoked VSD responses from primary barrel somatosensory cortex associated with the C2 whisker (BCS1), secondary barrel somatosensory cortex associated with the C2 whisker (BCS2) and from motor cortex associated with C2 whisker (mBC) indicating complete and spatially widespread inhibition of sensory-evoked activity in the cortex ( Supplementary Fig. 5 ). Having confirmed blockade of sensory-evoked activity in the cortex, we next examined the effect of TTX treatment on spontaneous infraslow activity observed from VSD imaging. We computed the magnitude of spontaneous infraslow activity in the cortex as the root mean square (RMS) value at each pixel location for 10 min of spontaneous infraslow VSD activity to generate a map of baseline infraslow activity ( Fig. 5a ). Following TTX treatment, the RMS values of infraslow spontaneous activity were attenuated throughout the cortex and the mean RMS of infraslow spontaneous activity was significantly reduced compared with untreated controls ( Fig. 5b ). Similarly, we repeated these experiments using antagonists of glutamatergic transmission, DNQX (500 μM) and AP5 (200 μM). Relatively high drug concentrations were required because of surface application and are consistent with blockade that we have achieved in the past [40] . Attempts to generate seed pixel correlation maps from residual spontaneous infraslow activity following treatment with TTX or DNQX and AP5 resulted in the absence of any functional structure even when presented as filled contour plots to guide visual analysis ( Fig. 5c ). 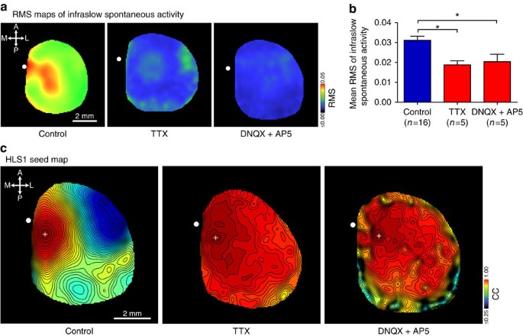Figure 5: Infraslow functional organization is disrupted by treatment with TTX and also by DNQX and AP5. (a) Root mean square (RMS) map of spontaneous infraslow activity under control conditions and following topical treatment with either TTX or DNQX and AP5. All RMS maps have been similarly scaled to the indicated colour bar. (b) Summary of the suppression of spontaneous infraslow activity. Mean RMS values derived from the entire imaged cortex for control (n=16), TTX-treated (n=5) and DNQX and AP5-treated (n=5) conditions. Error bars are s.e.m. *P<0.05, one-way analysis of variance, Bonferronipost hoc. (c). Functional correlation maps generated from infraslow spontaneous activity and depicted as filled contour plots under control conditions and following topical treatment with either TTX or DNQX and AP5. All correlation maps have been scaled to the indicated colour bar. Figure 5: Infraslow functional organization is disrupted by treatment with TTX and also by DNQX and AP5. ( a ) Root mean square (RMS) map of spontaneous infraslow activity under control conditions and following topical treatment with either TTX or DNQX and AP5. All RMS maps have been similarly scaled to the indicated colour bar. ( b ) Summary of the suppression of spontaneous infraslow activity. Mean RMS values derived from the entire imaged cortex for control ( n =16), TTX-treated ( n =5) and DNQX and AP5-treated ( n =5) conditions. Error bars are s.e.m. * P <0.05, one-way analysis of variance, Bonferroni post hoc . ( c ). Functional correlation maps generated from infraslow spontaneous activity and depicted as filled contour plots under control conditions and following topical treatment with either TTX or DNQX and AP5. All correlation maps have been scaled to the indicated colour bar. Full size image Neuroimaging of spontaneous infraslow activity has been the focus of tremendous research interest, but has typically relied upon imaging modalities that indirectly reflect neuronal activity [45] , [46] , [47] , [48] and have thus raised questions about the underlying nature and interpretation of these data [22] , [36] . Innovative efforts to directly assess the neurophysiological basis of fMRI BOLD signal fluctuations have revealed much about the best electrophysiological correlates of these signals, but these approaches require specialized recording equipment and technical analysis to remove electrical artifacts and are limited in their spatial coverage. In this study, we used VSD imaging to describe the spatiotemporal structure of spontaneous infraslow activity in anaesthetized mouse cortex. This approach allowed us to directly examine large, regional patterns of spontaneous electrical activity between and within cortical hemispheres and with high spatial and temporal resolution as well as allowing us to pharmacologically probe the mechanistic dependence of this activity. The use of VSD imaging is particularly advantageous for the investigation of infraslow functional connectivity for a number of reasons. The dye is a direct reporter of electrical activity in the brain with activity demonstrated to report neuronal membrane voltage in anaesthetized and awake mice [31] and whose neuronal activity dependence was probed by pharmacological intervention. The ‘blue’ oxonol dye, RH1692, is effectively excited at red wavelengths (630±15 nm) and emits fluorescence at wavelengths extending to the edge of the infrared spectrum (688±15 nm) thus greatly minimizing the potential for confounding signal artifacts associated with flavoprotein autofluorescence as well as intrinsic signals associated with haemodynamic response, breathing and heart rate [28] . Potential haemodynamic confounds arising from differential absorption of oxy-/deoxygenated haemoglobin in the VSD emission spectrum were experimentally tested using an activity-independent fluorescent probe and were found not to significantly contribute to our voltage signal ( Supplementary Fig. 6 ). These latter potential sources of signal contamination are thought to contribute to a global signal confound that accompanies imaging of infraslow activity in both fc-fMRI and intrinsic optical signal imaging [7] , [35] , [42] , [49] . Frequently, post-acquisition data processing to remove the global signal is implemented to reveal underlying functional connectivity, but remains controversial due to questions about the strictly artifactual nature of the global signal and the dependence of observed resting-state anti-correlations on its removal [35] , [50] . Although we did observe an increase in background correlation in infraslow spontaneous activity versus slow spontaneous activity, global signal removal was not necessary using VSD imaging to reveal infraslow functional connectivity. The dye also has an excellent signal-to-noise ratio and its efficacy has been established in monitoring sensory-evoked, optogenetically evoked and spontaneous activity at high spatial and temporal resolution [27] , [28] , [31] , [33] , [40] , [51] . We have previously demonstrated the high spatial resolution of our VSD imaging with an optical resolution of 67 μm (ref. 27 ). The fast temporal properties of the dye [28] , [52] also allow acquisition of spontaneous activity across multiple time scales [53] allowing the direct comparison of the functional structure of infraslow spontaneous activity and the cortical motif structures we have previously described using higher-frequency spontaneous activity as a source. This allows our comparative analysis to be internally controlled for factors such as surgical variability, anaesthetic brain state, and the precise registration of functional cortical regions of interest. We also demonstrate that imaging of the dye is stable for hours. We show that the VSD preparation is stable during the course of our experiments and during the long acquisition periods for spontaneous data collection ( Supplementary Fig. 2 ). This is consistent with our previous work indicating both stable sensory-evoked responses as well as stable cortical spontaneous EEG and VSD signal power following RH1692 dye loading [27] . We collected infraslow data under urethane-induced anaesthesia as it provided a stable brain state devoid of evoked or voluntary behavior, which might contaminate resting-state activity. Previous accounts of spontaneous, cyclic ultraslow transitions in cortical power (1.5–4 Hz) are not likely to be principal contributors to the infraslow functional organization described here, as we observe the persistence of this organization under light isoflurane (0.5%) anaesthesia and under awake states where such alternations are greatly reduced or absent [54] ( Supplementary Fig. 7 ). Also, previous evidence has suggested that infraslow resting-state networks persist across varied brain states including wakefulness, natural sleep and under anaesthetic states [5] , [9] . Consistent with this idea, we have demonstrated the persistence of cortical motif structure derived from both infraslow and slow spontaneous activity in both anaesthetized and quiet awake states [27] . The advent of increasingly sensitive genetically encoded voltage indicators (GEVI) [55] , [56] may permit future studies whereby long-duration awake state recordings may more readily be facilitated in combination with less invasive chronic imaging window preparations [57] , [58] . In addition, this strategy is advantaged by cell type-specific expression of the genetically encoded voltage indicators and the potential to minimize contaminating non-neuronal signals through a noise gain equalization of Förster resonance energy transfer signals [55] . We showed that infraslow spontaneous activity is heterogeneous and regional in nature. Infraslow activity is bilaterally synchronous with the highest degree of synchrony exhibited by midline areas such as aM2/AC, pM2 and RS cortices. These midline hotspots were consistent with previous results from our lab identifying highly correlated bilateral activity in these areas in higher-frequency spontaneous activity that was greatly attenuated in acallosal mice suggesting an important role for transcallosal fibres in mediating this synchrony [27] . Intriguingly, these structures are also consistent with cortical features recently described as components of the rat analogue of the DMN identified from fc-fMRI. In particular, prefrontal cortex and retrosplenial cortex were identified as hubs, comprising two distinct modules of the rat default network [6] . These results are also broadly similar to functional resting-state connectivity exhibited using intrinsic signal optical imaging, which reflects inherently infraslow processes in mice [7] and suggests common consistent features of infraslow, resting-state, bilateral connectivity across imaging modalities. We have previously examined mesoscale, intrahemispheric functional connectivity within higher-frequency spontaneous activity using VSD imaging to reveal recurrent, patterned regional activity called cortical motifs [33] . Using a seed pixel correlation analysis, we were able to investigate the activity structure of spontaneous infraslow activity. We demonstrated that infraslow spontaneous cortical activity exhibits an intrahemispheric activity structure that is strikingly similar to that of cortical motifs, characteristic patterned activity whose occurrence reverberates within slow spontaneous activity. Functional connectivity emanating from rodent retrosplenial cortex has features thought to be consistent with analogous connectivity from human DMN [6] . Interestingly, correlation maps generated from infraslow VSD activity recapitulated features of the rat DMN identified by fc-fMRI [6] . Noteworthy is the recruitment of medial cortices extending anteriorly toward, and encompassing aM2/CG. Consistent with rat fc-fMRI, this recruitment of medial cortices forms a band of connectivity described as a ‘medial ridge’ and is a feature distinct from the more focal, discontinuous midline connectivity described in the human DMN [6] . The similarity between infraslow and slow spontaneous cortical motifs is paralleled by observations from a study investigating the neurophysiological correlates of resting-state BOLD fluctuations in the cortices of a population of epileptic patients [10] . Here, the authors determined that the correlation structure of spontaneous activity from the slow cortical potential (<0.5 Hz), recorded from a large grid of electrocorticographic (ECoG) electrodes overlaid over sensorimotor cortex, exhibited a significant positive cross-correlation with the spatial pattern of activation for that area from a separately recorded resting-state fMRI session and that this relationship was apparent across awake, slow-wave sleep and REM states. Intriguingly, the correlation structure derived from 1–4 Hz spontaneous ECoG activity as well as gamma (50–100 Hz) band-limited power also positively correlated with the BOLD signal [10] . Similar observations of correlative spontaneous fluctuations in gamma LFP power as well as neuronal firing rates have been observed from simultaneous, bilateral recordings in auditory cortex [59] . However, it is the inference of analogous ECoG correlation structure between spontaneous activity derived from the slow cortical potential and from 1–4 Hz frequency activity that is consistent with our observation of the shared functional organization between infraslow and slow spontaneous VSD activity. In our approach, we are able to compare correlation maps generated not only from different frequencies of activity but also from the same source of spontaneous activity and thus reduce the potential for inconsistencies caused by uncontrolled variance that may arise from separately acquired resting states. Furthermore, we were not limited to only sensorimotor ROIs in our approach. The interconnected nature of the activity structure of infraslow and slow activity is consistent with a cross-frequency phase–amplitude coupling relationship that has previously been indicated for infraslow fluctuations in EEG and MEG recordings in human subjects [13] , [14] , [15] , [60] . In agreement with these studies, advancements permitting simultaneous localized neurophysiological measurements alongside fMRI indicate that changes in low-frequency (2–15 Hz) LFP and the slow modulation of gamma frequency LFP signals are strong neurophysiological correlates of activity for both evoked- and resting-state BOLD signal fluctuations in non-human primates [45] , [47] , [48] . Similar correlative findings between spontaneous infraslow (<0.1 Hz) frequency activity in LFP and resting-state BOLD signal have also been observed in anaesthetized rats [38] . These findings suggest that resting-state BOLD activity may thus reflect synaptic input and local cortical processing rather than neuronal output. VSD activity can indicate both super- and sub-threshold voltage activity but tends to correlate best with sub-threshold membrane potential changes [61] . As such, VSD imaging as performed in this study may be particularly apt at investigating infraslow fluctuations that may underlie similar processes related to spontaneous BOLD signal fluctuations. In our present study, we did not examine the activity structure of spontaneous gamma frequency activity as these signals lie at the detection limit of our imaging acquisition sampling rate. However, any residual gamma frequency activity is unlikely to have contributed to our functional mapping of spontaneous activity and would have been greatly attenuated by our filter processing. We show that infraslow correlation maps were abolished following acute pharmacological blockade of cortical voltage-gated sodium channels with TTX suggesting that the cortical functional connectivity exhibited in the infraslow frequency band is dependent on neuronal excitability ( Fig. 5c ). However, as TTX treatment alone has been demonstrated to be sufficient to block flavoprotein-dependent autofluorescence in rat somatosensory cortex [29] as well as blocking synchronous, infraslow large-scale astrocytic calcium waves [62] , we also examined the dependency of our observed infraslow activity on specifically excitatory glutamatergic transmission and found that DNQX and AP5 treatment also abolished infraslow functional organization ( Fig. 5 ). Residual infraslow RMS activity following pharmacological inhibition may represent the contribution from incomplete penetrance and blockade with our antagonists or also the contribution of persistent non-neuronal sources to fluctuations at this frequency ( Fig. 5a,b ). The inability to generate correlation maps exhibiting coherent functional organization from residual activity in this frequency band following treatment with antagonists is consistent with the latter interpretation, however, we cannot exclude the possibility that it may also reflect a distinct source of activity lacking this type of functional structure. Abolition of infraslow correlation maps was also accompanied by the substantial attenuation of spontaneous infraslow cortical power assessed by EEG ( Fig. 1e ) and by VSD imaging and provided confirmation that the underlying basis of our infraslow signals was truly neurophysiological. These results are significant as they provide a direct mechanistic link for infraslow signals and their observed functional connectivity that has not, to our knowledge, been previously demonstrated. Infraslow spontaneous activity has generated tremendous interest as a resource for revealing functional brain organization [3] , [18] , [63] . However, many questions remain regarding the neurophysiological basis of this activity. We report the activity structure of infraslow spontaneous activity using a direct reporter of electrical signals in the cortex and demonstrate its reliance upon cell excitability and glutamatergic signalling. The direct assessment of electrical brain activity and the adaptability of this experimental paradigm of neuroimaging of infraslow resting-state activity may provide a critical platform to probe mechanistic questions regarding the nature and function of infraslow activity in a manner that may synergistically complement concurrent ongoing fc-fMRI studies. Evidence suggesting that alterations in infraslow resting-state networks are associated with neurodegenerative disease processes has raised the potential of novel therapeutic biomarker identification [19] , [64] , [65] , [66] . Our data and approach in combination with the availability of animal models of neurodegenerative and psychiatric disease and the use of novel optogenetic tools from which to probe circuit and brain function may effectively compliment human clinical setting investigations and aid in increasing our understanding of the underlying basis of these networks and their pathological regional network dysfunction. Animals Adult (24–32 g) male C57BL6J mice aged 2–5 months were used for all the experiments ( n =37). Animals were housed in clear plastic cages in groups of two to five, under a 12:12 h light/dark cycle. Mice were given ad libitum access to water and standard laboratory mouse diet at all times. Animal protocols were approved by the University of British Columbia Animal Care Committee and were in accordance with guidelines set forth by the Canadian Council for Animal Care. Surgery For craniotomy surgery and for maintenance during imaging experiments, mice were anaesthetized with urethane as previously described [67] . Briefly, anaesthesia was induced with urethane (0.12% w/w) and body temperature was maintained at 37 °C with a heating pad and feedback regulation from a rectal temperature probe. Mice were placed on a metal plate that could be mounted onto the stage of the upright macroscope and the skull was fastened to a steel plate with cyanoacrylate glue and dental cement. A 8 × 8 mm unilateral craniotomy or bilateral craniotomy was made and the underlying dura was removed. Urethane-anaesthetized mice were tracheotomized to assist with breathing. VSD imaging For in vivo VSD imaging, the dye RH1692 (Optical Imaging, New York, NY), was dissolved in HEPES-buffered saline solution (1 mg ml −1 ) and applied to the exposed cortex for 60–90 min, staining all neocortical layers, as reported previously. VSD imaging began 30 min following washing unbound VSD. To minimize movement artifacts owing to respiration, the brain was covered with 1.5% agarose made in HEPES-buffered saline and sealed with a glass coverslip. For VSD data collection, 12-bit images were captured at 150 Hz sampling rate for sensory-evoked activity and at 20 Hz for spontaneous activity acquisition with a CCD camera (1M60 Pantera, Dalsa, Waterloo, ON) and EPIX E4DB frame grabber with XCAP 3.8 imaging software (EPIX, Inc., Buffalo Grove IL). VSD was excited with a red LED (Luxeon K2, 627 nm centre) and excitation filters 630±15 nm as described. Images were taken through a macroscope composed of front-to-front video lenses (8.6 × 8.6 mm field of view, 67 μm per pixel). The resolution along the optical axis of our imaging setup was ∼ 1 mm (ref. 40 ). VSD fluorescence was filtered using a 673–703-nm bandpass optical filter (Semrock, New York, NY). As animal brain states exhibit spontaneous change, we averaged 10 trials of stimulus presentation to reduce these effects. To correct for time-dependent changes in VSD signals that accompany all imaging, we also collected a number of non-stimulation trials that were used for normalization of stimulated data. A 10-s interval between each sensory stimulation was used. To reduce potential VSD signal distortion caused by the presence of large cortical blood vessels, we focused into the cortex to a depth of ∼ 1 mm. To reduce regional bias in VSD signal caused by uneven dye loading or due to brain curvature, all VSD responses were expressed as a per cent change relative to baseline VSD responses (Δ F / F 0 × 100%) using custom-written code in Matlab (Mathworks, Natick, MA). VSD imaging of spontaneous activity was performed in the absence of visual, olfactory, tactile or auditory stimulation during 30 min epochs with 50 ms (20 Hz) temporal resolution. Ambient light resulting from VSD excitation (630 nm) was measured at 8.65 × 10 −3 W m −2 . Total duration of VSD excitation in a typical imaging experiment ranged from 900–1,200 s. VSD Δ/ F 0 (%) and cortical EEG power were stable during image acquisition and indicated little phototoxicity under the conditions we used. The fluorescence changes were quantified as ( F − F 0 )/ F 0 × 100 where F represents the fluorescence signal at any given time and F 0 represents the average of fluorescence over all frames. Awake VSD imaging Young (8–10 weeks old) male mice ( n =7) were surgically implanted with a screw on the skull for immobilization to a fixed connector. After 7 days for recovery, mice were habituated as previously described [27] , [33] in a modified plastic body chamber. Following habituation, craniotomy surgery and RH1692 labelling was performed under isoflurane anaesthesia (0.5–2% maintenance mixed with oxygen). Following surgery, mice were maintained under light isoflurane anaesthesia (0.5%) and pre-imaging of anaesthetized spontaneous activity was acquired. Isoflurane was then removed and mice were revived in place. Body temperature was maintained during revival by a heating pad placed underneath the body chamber. Acquisition of VSD imaging of spontaneous activity was initiated 10–50 min following removal from isoflurane anaesthesia, and data acquisition continued for an additional 40–60 min. Confirmation of awake status was obtained by synchronous recording of behavioural video (Raspberry Pi camera module) under infrared illumination, and also from EMG recordings from an electrode (cut acupuncture needle; 0.14 mm diameter) placed in muscle at the back of the neck. Buprenorphine was injected (0.075 mg kg −1 body weight intraperitoneally) 24 h before data acquisition to provide pre-surgical analgesia. In the course of recordings, mice appeared relatively unstressed and intermittently exhibited normal behaviours including attempted locomotion, chewing, licking, whisking and posture adjustments. These periods of active normal behaviours were identified by video and EMG recordings and were removed from our video epochs of spontaneous activity used for analysis of quiet wakefulness [33] . Following acquisition of awake imaging, mice were re-anaesthetized in place with isoflurane (0.5%) and cortical mapping via sensory stimulation was obtained. Cortical EEG recording A Teflon-coated, chloridized silver wire (0.125 mm) was placed on the right or left edge of the craniotomy. A reference electrode was placed on the nasal bone. The cortical signal was amplified ( × 1,000) and low-pass filtered (1,000 Hz) using a DAM 50 amplifier (World Precision Instruments). LFP recording Glass micropipettes with resistances between 4 and 6 MΩ were used for recording local field potential. The LFP signal was amplified ( × 1,000) and low-pass filtered (1,000 Hz) using a Multiclamp 700A (Molecular Devices) amplifier and digitized using a 1322A Digidata digitizer. Sensory stimulation Sensory stimuli were used to generate maps of sensory cortical areas and to provide reference locations from which to derive functional defined cortical ROIs. We used forelimb, hindlimb, whisker, visual and auditory stimulation. To stimulate forelimb and hindlimb, thin acupuncture needles (0.14 mm) were inserted into the paws and a 0.2–1 mA, 1 ms electrical pulse was delivered. To stimulate a single whisker (C2), the whisker was isolated and attached to a piezoelectric device (Q220-A4-203YB, Piezo Systems, Inc., Woburn, MA), and given a single 1 ms tap using a square pulse. The whisker was moved ∼ 90 μm in an anterior-to-posterior direction corresponding to a 2.6° angle of deflection. A 1 ms pulse of combined green and blue light delivered from a closely positioned LED was used as visual stimulation. A single 1 ms tone (25 kHz) was used as auditory stimulation. Averages of sensory stimulation were calculated from 10 trials of stimulation with an interstimulus interval of 10 s. Data analysis Sensory stimulation was used to determine the coordinates for the primary sensory areas (HLS1, FLS1, BCS1, V1 and A1), secondary somatosensory areas (HLS2, FLS2 and BCS2) and primary motor cortex for whisker. From these primary sensory coordinates, the relative locations of additional association areas were estimated using stereotaxic coordinates (ptA, RS, M2, V2MM, V2L, mHL and mFL). Infraslow (0.02–0.08 Hz) and slow (0.5–6.0 Hz) spontaneous VSD activity were isolated offline following data acquisition. Slow spontaneous activity was analysed as previously described [27] , [33] . Spontaneous VSD activity was integrated to a 1 Hz sampling rate and the resultant activity was then digitally passband filtered using zero-phase lag Chebyshev bandpass filter (zero-phase filter) at 0.02–0.08 Hz. In both the cases, a Chebyshev Type I filter design was used with a filter order of four and eight poles. To create seed pixel correlation maps, we calculated the zero-lag Pearson product–moment correlation between the VSD signal time course extracted from a seed pixel of interest and every pixel within the imaging area. The length of activity used to calculate the correlation index was 30 min for infraslow and slow spontaneous activity. Pharmacology For pharmacological experiments, the cortex was covered with HEPES-buffered saline solution to allow for later topical application of 10 μM TTX, a fast voltage-gated, sodium channel blocker. For experiments using DNQX (200 μM) and AP5 (500 μM), stock drug concentrations were dissolved in DMSO with a final concentration 0.4% DMSO present during experiments. Vehicle control experiments included 0.4% DMSO dissolved in HEPES-buffered saline solution. For all pharmacological experiments and controls, drugs were applied to the cortex for 30 min before imaging acquisition recommenced. Following incubation of drugs, 1.5% agarose made in HEPES-buffered saline was poured over the cortex and sealed with a glass coverslip to reduce movement artifacts during imaging. To maintain antagonist exposure during imaging, drugs were additionally diluted into molten agarose. Due to the long duration of imaging experiments and incubations, drug washout was not attempted. Importantly sham drug application was used for comparison and to control against nonspecific time-dependent effects. TTX and glutamatertigic receptor antagonist treatment in this manner previously blocked cortical activity in all the layers [68] , [69] . Statistics Spatial correlation analysis . As previously described [27] , we computed seed pixel correlation maps using temporal correlation of data obtained from spontaneous infraslow and spontaneous slow activity for multiple cortical regions for each animal. We compared sets of these seed pixel correlation maps using spatial correlation analysis within the animals (examining how relative patterns change within a subject), which removes the necessity of registration and alignment across animals. ‘Sets’ were defined as seed pixel correlation maps generated from the same seed pixel location (for example, HLS1) and by the origin of the activity from which the maps were generated (infraslow spontaneous activity versus slow spontaneous activity) for each animal. We observed that some sets are relatively homogeneous (by the same seed pixel location but obtained from different origins of activity) and distinct from other sets (by different seed pixel locations, but obtained from the same source of activity). In this case, the statistical significance of these comparisons depended on how consistent the individual spatial correlations were within a set and how different they were between sets. To determine statistical significance across animals, we calculated t-statistics for each comparison of one set of correlation maps with another set of correlation maps, computed using spatial correlation analysis in an identical fashion from different data (different sets across animals). For these analyses, the degrees of freedom are constrained by the number of experimental replicates (number of mice) used for comparisons under the same experimental conditions. To minimize the local contribution of correlation values around the seed pixel in spatial correlation analysis, we used a two-dimensional Gaussian fit to create a template image for each individual correlation map that models the local distribution of the correlation values centred around the seed pixel. To exclude the contribution of the first-order local correlations, we subtracted the template image from its corresponding original map. The resulting residual map contained only the second-order long-range correlation. The exclusion zone often encompass several millimetres in size (See Supplementary Fig. 4 ). We used these residual maps in our group data correlation analysis between maps obtained from infraslow and slow spontaneous activity. Error bars and±ranges represent standard error. *, **, *** and **** denote P <0.05, P <0.01, P <0.001 and P <0.0001, respectively. All the statistical tests were two-sided. How to cite this article: Chan, A.W. et al. Mesoscale infraslow spontaneous membrane potential fluctuations recapitulate high-frequency activity cortical motifs. Nat. Commun. 6:7738 doi: 10.1038/ncomms8738 (2015).